Near-infrared-featured broadband CO2reduction with water to hydrocarbons by surface plasmon 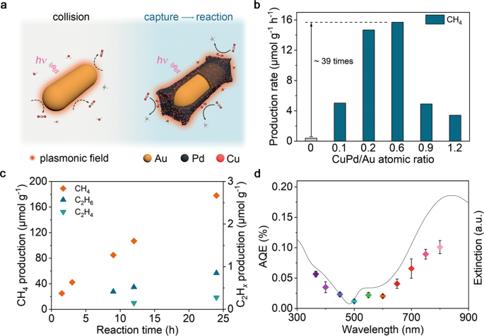Fig. 1: Plasmon-induced CO2RR performance. aSchematic illustration of the role of CuPd co-catalyst in capturing CO2molecules. Plasmonic catalysis usually takes place very close to the catalyst surface (i.e., within the range of the plasmon-induced local field). For the pure Au nanorods, the probability of the pure Au nanorods and CO2molecules to contact through the collision is very low (left), resulting in low CO2conversion efficiency. For the Au rod@CuPd, CuPd co-catalyst can capture CO2molecules and enhance the CO2concentration on the catalyst surface, increasing the opportunity for their further activation and conversion (right).bAverage production rates of CH4over Au rod@CuPd2with different shell thicknesses.cTime-dependent CH4production over Au rod@CuPd2in 24 h.dCalculated AQEs (color dots) over Au rod@CuPd2under different monochromatic light illumination, in reference to its UV-vis extinction spectrum (black line). The error bars represent the standard deviation of the experiments. The catalytic experiments of (b,c) are all carried out in CO2-saturated water and CO2atmosphere without any sacrificial agent under 400 mW cm–2full-spectrum light illumination. Imitating the natural photosynthesis to synthesize hydrocarbon fuels represents a viable strategy for solar-to-chemical energy conversion, where utilizing low-energy photons, especially near-infrared photons, has been the ultimate yet challenging aim to further improving conversion efficiency. Plasmonic metals have proven their ability in absorbing low-energy photons, however, it remains an obstacle in effectively coupling this energy into reactant molecules. Here we report the broadband plasmon-induced CO 2 reduction reaction with water, which achieves a CH 4 production rate of 0.55 mmol g −1 h −1 with 100% selectivity to hydrocarbon products under 400 mW cm −2 full-spectrum light illumination and an apparent quantum efficiency of 0.38% at 800 nm illumination. We find that the enhanced local electric field plays an irreplaceable role in efficient multiphoton absorption and selective energy transfer for such an excellent light-driven catalytic performance. This work paves the way to the technique for low-energy photon utilization. Artificial photosynthesis offers an appealing way to store intermittent solar energy by directly converting CO 2 , H 2 O and sunlight into hydrocarbon compounds [1] , [2] , [3] , [4] . Therewith, a myriad of semiconductors and metal nanocatalysts have been studied, demonstrating their feasibility in light-driven CO 2 reduction reaction (CO 2 RR) [5] , [6] , [7] . Nonetheless, the low utilization efficiency of the solar spectrum, especially the low-energy photons, and the sluggish process for energy coupling into the reactant molecules are the two critical obstacles that limit their further expansion toward technoeconomic applications. Moreover, the selective production of high-energy-value hydrocarbons involving multiple electron-proton transfer steps through CO 2 RR is another great challenge constraining their potential [8] . Plasmonic metal nanoparticles exhibit strong interaction with incident light in the form of localized surface plasmon resonance (LSPR) [9] , [10] . The absorption wavelength center of such LSPR can be easily tuned from ultraviolet (UV) to near-infrared (NIR) range just by changing the geometry structure (including symmetry, size, etc.) of plasmonic nanomaterials [11] , [12] , allowing them to have the wide possibility as light-harvesting units for solar-to-chemical energy conversion [13] , [14] , [15] , [16] , [17] , [18] , [19] . Recently, it was demonstrated that specific plasmonic nanostructures are able to convert CO 2 under laser irradiation with the help of organic additives [20] , [21] , suggesting their potential in CO 2 RR. In addition, the rates of plasmon-induced catalytic reaction exhibit a super-linear power law dependence on the number of incident photons, providing a positive relationship between quantum efficiency and photon flux [22] . Amidst the fascinating development of such plasmonic materials, it is discovered that the mismatch of quick LSPR relaxation (up to ~100 ps) and slow chemical reduction kinetics (several milliseconds or seconds) in time scale severely retards the conversion efficiency of solar energy [23] , [24] , [25] . To break this bottleneck, versatile co-catalysts are employed to establish an effective bridge for transferring hot carriers from plasmonic materials into reactant molecules [13] , [14] , [15] , [16] , [17] , [26] . In this respect, the precise design of the co-catalyst toward efficient hot carrier accepting ability and unique CO 2 chemisorption capability is highly sought. Here we employ Au rod as a plasmonic light-harvesting unit and copper-palladium (CuPd) alloy shell as a co-catalyst to realize efficient plasmon-induced artificial photosynthesis in the absence of the additional sacrificial agent, achieving nearly 100% CH 4 product selectivity under full-spectrum light illumination. As deciphered by in situ near ambient pressure X-ray photoelectron spectroscopy (NAP-XPS) and density functional theory (DFT) calculations, the localized electric field, which leads to the emergence of a new isolated state above the Fermi energy ( E f ) and the differentiation of electron transfer within different molecular orbitals, enables such a unique solar-to-chemical energy conversion. By optimizing the reaction system, an impressive CH 4 production rate of 0.55 mmol g −1 h −1 is achieved via a gas-solid biphase system, demonstrating a record-high apparent quantum efficiency (AQE) of 0.38% at 800 nm NIR light illumination. Plasmon-induced CO 2 reduction with water The CuPd co-catalyst can capture CO 2 molecules and enhance the CO 2 density on the catalyst surface, which allows the reactants to locate within the range of the plasmon-induced local field, increasing the opportunity for their further activation and conversion (see Fig. 1a ). Typically, we obtain the Au rod@CuPd core-shell composites via a wet chemical synthesis (Fig. S 1 ). The shell thickness and Pd/Cu ratio of the Au rod@CuPd core-shell composites can be easily controlled by changing the amount of metal precursors (see Tables S1 , S2 , and Figs. S2 – S5 for the list of prepared samples). Taking Au rod@CuPd 2 as an example, the transmission electron microscopy (TEM) image (Fig. S 3a ) shows that the rod structure is preserved after the deposition of the CuPd shell onto the Au surface. The fast Fourier transform patterns and magnified images of the selected area in Fig. S 6, a,b , are well-fitted with a pure face-centered cubic crystal structure viewed along the [110] and [100] directions, respectively. The ordered lattice fringes with a spacing of 2.35 and 2.05 Å are attributed to the (111) and (002) planes of Au lattice, respectively, indicating that precursor ions are epitaxially reduced on the surface of Au rods to form a CuPd single-crystal shell. Such a result can be also supported by the X-ray diffraction (XRD) analysis (Fig. S 7 ) and the elemental mapping profiles (Fig. S 8 ). In addition, the Pd and Cu K-edge X-ray absorption near-edge structure (XANES, Fig. 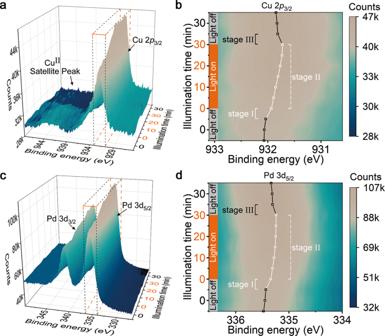Fig. 2: Deciphering plasmon-induced electron behavior via in situ NAP-XPS characterization. aandbIn situ NAP-XPS spectra of Cu 2p3/2(a) and contour plot for the amplified top view of the selected box-shaped area (b).c,dIn situ NAP-XPS spectra of Pd 3d5/2(c) and contour plot for the amplified top view of the selected box-shaped area (d). The in situ NAP-XPS data are recorded continuously for 1 h over Au rod@CuPd2at 0.25 mbar CO2atmosphere and light illumination is introduced into the catalytic system in the middle 30 min (marked in orange color). Representative peak positions are marked with open squares in (b) and (d). The squares and lines in black and white indicate unilluminated and illuminated conditions, respectively. S 9 ) and Fourier transformed extended X-ray absorption fine structure (EXAFS, Fig. S 10 ) spectra of the prepared samples show that the total coordination numbers of Pd and Cu are smaller than 12 (see Table S3 ), further confirming that the Pd and Cu elements are located in the outermost shell of these samples. Then we employ UV-vis extinction spectra to evaluate the light-harvesting ability of the prepared samples. As shown in Fig. S 11 , two peaks around 510 and 740 nm are the typical characteristics of the transversal and longitudinal LSPR modes of Au nanorod, respectively [27] , [28] . It is discovered that, compared with the Cu/Pd molar ratio, the CuPd thickness has a more prominent influence on the optical properties, allowing the remarkable broadening of the absorption range of prepared samples into the NIR region. Fig. 1: Plasmon-induced CO 2 RR performance. a Schematic illustration of the role of CuPd co-catalyst in capturing CO 2 molecules. Plasmonic catalysis usually takes place very close to the catalyst surface (i.e., within the range of the plasmon-induced local field). For the pure Au nanorods, the probability of the pure Au nanorods and CO 2 molecules to contact through the collision is very low (left), resulting in low CO 2 conversion efficiency. For the Au rod@CuPd, CuPd co-catalyst can capture CO 2 molecules and enhance the CO 2 concentration on the catalyst surface, increasing the opportunity for their further activation and conversion (right). b Average production rates of CH 4 over Au rod@CuPd 2 with different shell thicknesses. c Time-dependent CH 4 production over Au rod@CuPd 2 in 24 h. d Calculated AQEs (color dots) over Au rod@CuPd 2 under different monochromatic light illumination, in reference to its UV-vis extinction spectrum (black line). The error bars represent the standard deviation of the experiments. The catalytic experiments of ( b , c ) are all carried out in CO 2 -saturated water and CO 2 atmosphere without any sacrificial agent under 400 mW cm – 2 full-spectrum light illumination. Full size image Upon having a comprehensive understanding of the structural information and optical properties of the Au rod@CuPd, we assess their efficacy for CO 2 RR in a conventional reactor consisting of CO 2 -saturated water and suspended catalysts (see Fig. S12 ). After continuous illumination for 3 h, only CH 4 can be detected with a maximum production rate of 15.6 μmol g −1 h −1 , ca. 39 times that of Au rod, demonstrating the excellent catalytic performance of Au rod@CuPd 2 (Fig. 1b ). The production rates of CH 4 show a volcano-shaped relationship with the CuPd/Au ratios, which can be attributed to the competition of increased surface active sites and aggravated electron-phonon scattering in the thickened CuPd shell [16] . The linear time-dependent CH 4 production shown in Fig. 1c corroborates the excellent durability of Au rod@CuPd 2 . Moreover, C 2 H 6 and C 2 H 4 can also be detected after the long-term test, suggesting the presence of multiple proton-coupled electron transfer processes during the reaction, which is uncommon in conventional photocatalysis. In the meantime, after normalizing the CH 4 production rates by the amount of Cu (orange dots in Fig. S 13 ), the catalytic performances of samples with different Cu/Pd atomic ratios are similar, suggesting the inseparable role of Cu in CO 2 RR. The wavelength-dependent apparent quantum efficiencies (AQEs), which are in good agreement with the extinction spectrum of Au rod@CuPd 2 , are up to 0.1% at 800 nm (see Fig. 1d ). This result explicitly suggests the unique features of Au rod@CuPd 2 in effectively utilizing low-energy photons in the absence of the sacrificial agent (see also Fig. S 14 ). In cyclic tests under 800 nm monochromatic light illumination, the production rates of CH 4 are well maintained for 10 runs (each run for 3 h, Fig. S 15 ), verifying the long-term stability of Au rod@CuPd 2 . Furthermore, hydroxyl radicals ( • OH) are detected as the main oxidative product by electron spin resonance spectroscopy (Fig. S 16 ). The verification of product origin is another key aspect. The conditions for various control experiments and corresponding results are illustrated in Fig. S 17 (see also Table S4 for details). Unambiguously, catalyst, light, CO 2 and H 2 O are keys for CO 2 RR over Au rod@CuPd 2 and the CH 4 can hardly be produced from the direct photolysis or pyrolysis of the carboneous compounds (e.g., surfactants and reducing agents for catalyst synthesis). We further employ synchrotron radiation vacuum UV photoionization mass spectrometry (SVUV-PIMS) to convincingly identify the origin of the CH 4 product. As shown in Fig. S 18, a,b , the peaks at m/z = 16 and 17 can be assigned to 12 CH 4 and 13 CH 4 when using 12 CO 2 and 13 CO 2 as the feed gas, respectively, firmly suggesting that the CO 2 feed gas is indeed the carbon source of produced CH 4 . In addition, we employ offline sum frequency generation vibrational spectroscopy (SFG-VS) to monitor the surface intermediates formed during the photocatalytic reaction. As shown in Fig. S 19, a,b , after illumination for 5 min, three SFG-VS signals appear at 2880, 2945, and 2965 cm −1 , which can be assigned to the symmetric stretching (ν s C–H), Fermi-resonance (ν Fermi C–H) and asymmetric stretching (ν as C–H) modes of the generated methyl groups, respectively [29] . This observation firmly demonstrates the evolution of CO 2 and H 2 O to methyl groups at the catalytic interface. Mechanism for plasmon-induced catalytic process The direct charge transfer mechanism provides a reasonable explanation for the unique selectivity in plasmon-induced catalytic process [30] , [31] , [32] . Nevertheless, in the case of our work, a critical issue is that the energy of a single low-energy photon (~1.55 eV for 800 nm light) is insufficient for reaching the energy barrier of CO 2 RR without adding sacrificial agent. To gain insight into such a low-energy photon utilization ability for CO 2 RR, we employ in situ NAP-XPS to examine the plasmon-induced light-matter interaction in the catalytic system. All NAP-XPS spectra have been calibrated with the Au 4 f core level of Au foil, which is mounted beside the sample (see Fig. S 20 ). Under the dark condition, no obvious fluctuation arises in the binding energy of Cu (Fig. 2a, b ). Once turning on the light, the binding energy of the Cu peak instantaneously decreases (Stage I), and then is gradually reduced (Stage II) under subsequent light illumination. When the light is turned off, the binding energy of Cu increases immediately (Stage III) but cannot return to the initial level. Based on these observations, we can infer that the changes in Cu involve two conceivable processes, where one is fast and reversible (Stage I and III), and the other is slow and irreversible (Stage II). For Stage I and III, electron energy fluctuation appears when the interaction of incident light with catalyst changes. This phenomenon can be attributed to the accumulation of hot electrons above the Fermi level ( E f ), whose lifetime typically lasts only a few hundred femtoseconds [24] , [33] . For Stage II, it is accompanied by the gradual disappearance of the Cu II satellite peak in Fig. 2a , suggesting that the Cu elements are gradually reduced under light illumination by the hot electrons generated by LSPR relaxation (see also Figs. S21 and S22 ). Such a chemical state change is relatively sluggish and can be responsible for the slow process. By analyzing the changes of Pd 3 d NAP-XPS spectra in Fig. 2c, d , we can confirm that Pd shows similar three-stage behavior to Cu 2 p 3/2 . 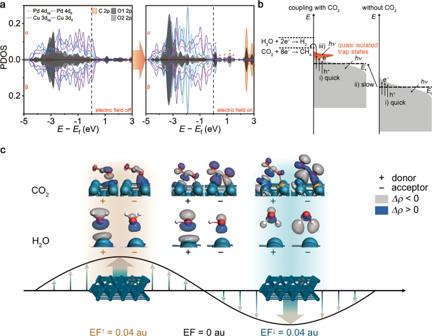Fig. 3: Theoretical calculations: the key role of local field in multiphoton absorption and energy transfer processes. aThe projected density of states (PDOS) of CO2adsorbed on a CuPd (100) surface in the absence (left) and presence (right) of electric field pointing toward the surface. The main quasi isolated trap states are marked with orange asterisks.bSchematic illustration for the plasmon-induced energy transfer in CO2RR, where they-axis is energy (E) and the gray shading indicates filled electronic states. Three key processes for initiating and enhancing the plasmon-induced CO2RR include (i) fast excitation and accumulation of electrons above the Fermi level (Ef), (ii) plasmon-induced slow photoreduction of Cu and Pd, and (iii) formation of new isolated trap state (origin shading) by coupling CO2molecule with metal orbitals and re-excitation of the electrons above the Fermi level, which eventually result in the CO2RR process.cNOCV orbitals relevant to the most important deformation density in CO2and H2O on a CuPd (100) surface in the absence (middle column) and presence of electric field toward (right column) or away from (left column) the surface. Donor NOCV on the left and acceptor NOCV on the right are displayed in each panel. Isovalue is set to 0.015. 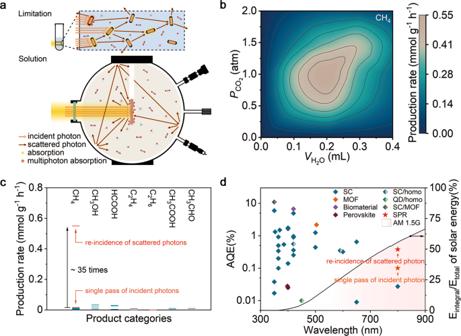Fig. 4: Optimized plasmonic catalysis: efficient utilization of scattered photons. aSchematic illustration of the gas-solid reaction, where mixed vapor of CO2and H2O with centrally installed catalyst nanoparticles contained in a spherical reactor is illuminated with full-spectrum light. During the reaction, the scattered photons can be reflected to the catalyst surface, leading to efficient multi-absorption processes.bAverage production rates of CH4through plasmon-induced CO2RR using the gas-solid reaction device over Au rod@CuPd2under different CO2pressure and H2O volume. The catalytic experiments are carried out in the mixed vapor of CO2and H2O without any sacrificial agent under 400 mW cm–2full-spectrum light illumination.c,dThe comparison of production rates (c, see TableS5) and AQEs (d, see TableS6) of Au rod@CuPd2reported in this work with the records reported in the literature for the last 5 years on artificial photosynthesis, which directly convert CO2, H2O and sunlight into compounds without sacrificial agent. From the viewpoint of catalysis, the slow photoreduction and the fast hot-electron accumulation above the E f are both beneficial to improve the chemical potential of the catalyst [34] , [35] , which is vital to break its catalytic limitation. In the meantime, we also monitor the C 1 s spectra through in situ characterization. As shown in Fig. S 23 , two peaks at 284.4 and 293.2 eV attributed to the adsorbed C species (C ad species) and gaseous CO 2 (g-CO 2 ), respectively, can be observed. The relative increase in peak area (see Fig. S 21 ) and positive shift of the binding energy of g-CO 2 peak under light conditions represent the continuous adsorption of CO 2 molecules and their conversion process to hydrocarbons [36] , [37] , [38] . Fig. 2: Deciphering plasmon-induced electron behavior via in situ NAP-XPS characterization. a and b In situ NAP-XPS spectra of Cu 2 p 3/2 ( a ) and contour plot for the amplified top view of the selected box-shaped area ( b ). c , d In situ NAP-XPS spectra of Pd 3 d 5/2 ( c ) and contour plot for the amplified top view of the selected box-shaped area ( d ). The in situ NAP-XPS data are recorded continuously for 1 h over Au rod@CuPd 2 at 0.25 mbar CO 2 atmosphere and light illumination is introduced into the catalytic system in the middle 30 min (marked in orange color). Representative peak positions are marked with open squares in ( b ) and ( d ). The squares and lines in black and white indicate unilluminated and illuminated conditions, respectively. Full size image To reveal the mechanism how CO 2 is activated with the catalyst upon light irradiation, we further investigate the key role of unoccupied adsorbate states, by analyzing the projected density of states (PDOS, Fig. 3a ) of our catalytic system consisting of catalyst and CO 2 molecule. With CuPd as catalytic sites, the CO 2 molecule can form hybrid states with the catalyst upon adsorption. Upon introduction of the electric field to the hybrid states, the calculation indicates that the state peaks of O1 2 p and O2 2 p shift toward lower energy and form a larger overlap area with the more localized Pd 4 d z and Cu 3 d z (parallel to the electric field) states, enhancing the stability of the key adsorption configuration [39] . More importantly, a series of new quasi isolated trap states emerge above the E f in the presence of the electric field as illustrated in Fig. 3a . Compared to the continuous states near E f of PdCu metal, these quasi isolated trap states can effectively extend the lifetime of hot electrons and increase the probability of electron re-excitation by another low-energy photon [40] , [41] , which makes the utilization of low-energy photons possible. Such a multiphoton absorption behavior can be corroborated by the superlinear law dependence between CH 4 production rate and light intensity (see Figs. S24 – S27 ) [19] , [20] , [22] . Taken together, the information gleaned by NAP-XPS and theoretical calculation can put forward the mechanism for plasmon-induced charge transfer in CO 2 RR as shown in Fig. 3b . Generally, there are three key processes for initiating and enhancing the plasmon-induced CO 2 RR, including (i) fast excitation for accumulating hot electrons above the Fermi level ( E f ), (ii) slow photoreduction process for elevating the chemical potential of the catalytic sites, and (iii) emergence of new quasi isolated trap states for re-exciting the electrons, gaining sufficient energy for triggering CO 2 RR. During the light-driven CO 2 RR, the three distinct processes work together to realize the utilization of low-energy NIR light for the reaction. Fig. 3: Theoretical calculations: the key role of local field in multiphoton absorption and energy transfer processes. a The projected density of states (PDOS) of CO 2 adsorbed on a CuPd (100) surface in the absence (left) and presence (right) of electric field pointing toward the surface. The main quasi isolated trap states are marked with orange asterisks. b Schematic illustration for the plasmon-induced energy transfer in CO 2 RR, where the y -axis is energy ( E ) and the gray shading indicates filled electronic states. Three key processes for initiating and enhancing the plasmon-induced CO 2 RR include (i) fast excitation and accumulation of electrons above the Fermi level ( E f ), (ii) plasmon-induced slow photoreduction of Cu and Pd, and (iii) formation of new isolated trap state (origin shading) by coupling CO 2 molecule with metal orbitals and re-excitation of the electrons above the Fermi level, which eventually result in the CO 2 RR process. c NOCV orbitals relevant to the most important deformation density in CO 2 and H 2 O on a CuPd (100) surface in the absence (middle column) and presence of electric field toward (right column) or away from (left column) the surface. Donor NOCV on the left and acceptor NOCV on the right are displayed in each panel. Isovalue is set to 0.015. Full size image Given the key role of hybrid states in the mechanism, we further look into the hybrid orbitals composed of catalytic sites and CO 2 or H 2 O molecules through DFT calculations. The optimized geometries and adsorption energies of molecules on CuPd (100) surface in different field conditions are illustrated in Fig. S 28 . Although the electron transfers from CuPd (100) surface to H 2 O and CO 2 molecules exhibit similar trends (see Fig. S 29 ), the CO 2 and H 2 O display different natural orbitals for chemical valence (NOCVs) (Fig. 3c ). In detail, when electric field points toward the metal surface, the electrons of CO 2 are redistributed from O lone-pair orbital to its antibonding π* orbital, weakening the C–O bond and increasing the bond length. When the electric field points away from the metal surface, the lone-pair electrons transfer to the σ orbital between O and the metal atom. However, the electron transfer in adsorbed H 2 O molecules only oscillates between the bonding orbital of H 2 O and the orbital of Pd atoms. Thus the electric field provides scant assistance to the cleavage of the O–H bond. Based on these results, it is confirmed that the local electric field can facilitate the directional electron transfer to CO 2 molecules, which contributes to the selective production of hydrocarbons. Performance enhancement based on catalytic mechanism Upon demonstrating the opportunity of utilizing low-energy photons in plasmon-induced CO 2 RR, it remains an open question whether it is possible to further improve the photon utilization for enhanced multiphoton absorption. Given the super-linear relationship between plasmonic catalytic rate and photon flux (i.e., the light intensity, Fig. S 26 ), the inevitable scattering loss of incident light becomes the main limitation of the conventional reaction system (see Fig. 4a ). To overcome the limitation, we design a gas-solid reaction system with a spherical structure to realize the re-incidence of scattered photons, which works only for the plasmonic catalytic system rather than conventional photocatalysis. By optimizing the volume of H 2 O and the partial pressure of CO 2 , the CH 4 production rate of the light-driven CO 2 RR performed in such a system reaches 0.55 mmol g −1 h −1 (7.5 mmol g Cu −1 h −1 ) under 400 mW cm −2 full-spectrum light illumination (Fig. 4b ), ca. 35 times higher than that in the reaction system allowing only a single pass of the incident photon. To verify the catalytic nature, turnover number (TON) is calculated (see Supplementary Text for detail). A TON of 9.6 per exposed Cu atoms is obtained after 3 h of illumination given that no catalyst deactivation has been observed in long-term operation. In the meantime, the control experiments are also performed in the dark at an elevated temperature (see Fig. S 30 and Table S5 ), which matches the local temperature on the surface of catalyst nanoparticles under photoexcitation, to confirm the indispensability of light illumination. This conversion rate, enabled by the reaction system design taking advantage of plasmonic catalysis mechanism, far exceeds the current literature record (Fig. 4c and Table S6 ). Notably, the AQE in the gas-solid reaction at 800 nm is promoted to 0.38%. Such a superior photoconversion efficiency under low-energy NIR light illumination, which is even comparable with the efficiencies of the representative works in CO 2 RR with high-energy photons, allows our Au rod@CuPd 2 catalyst to hit the record-high CO 2 RR AQEs under NIR light illumination (Fig. 4d and Table S7 ). Fig. 4: Optimized plasmonic catalysis: efficient utilization of scattered photons. a Schematic illustration of the gas-solid reaction, where mixed vapor of CO 2 and H 2 O with centrally installed catalyst nanoparticles contained in a spherical reactor is illuminated with full-spectrum light. During the reaction, the scattered photons can be reflected to the catalyst surface, leading to efficient multi-absorption processes. b Average production rates of CH 4 through plasmon-induced CO 2 RR using the gas-solid reaction device over Au rod@CuPd 2 under different CO 2 pressure and H 2 O volume. The catalytic experiments are carried out in the mixed vapor of CO 2 and H 2 O without any sacrificial agent under 400 mW cm –2 full-spectrum light illumination. c , d The comparison of production rates ( c , see Table S5 ) and AQEs ( d , see Table S6 ) of Au rod@CuPd 2 reported in this work with the records reported in the literature for the last 5 years on artificial photosynthesis, which directly convert CO 2 , H 2 O and sunlight into compounds without sacrificial agent. Full size image This work emphasizes the irreplaceable role of plasmon-induce local fields in the solar-to-chemical energy transfer process, providing a riveting picture of the potential of plasmon-induced catalysis toward achieving broadband artificial photosynthesis, particularly with the utilization of low-energy photons, and renders new insights for pushing forward the future development of plasmonic catalysis. Such a technique for low-energy photon utilization can potentially be integrated with the existing techniques available for UV and visible light in the future. Materials Potassium(II) tetrachloropalladate (K 2 PdCl 4 , 99.99%) was obtained from Beijing HWRK Chem Co., LTD. Sodium borohydride (NaBH 4 , 98%) was obtained from Sigma Aldrich. 13 CO 2 isotope was obtained from Sigma Aldrich. Copper(II) chloride dihydrate (CuCl 2 ·2H 2 O) was obtained from Aladdin. Gold(III) chloride tetrahydrate (HAuCl 4 ·4H 2 O, 99.95%), ascorbic acid (AA, 99.7%), hexadecyl trimethyl ammonium bromide (CTAB, 99.0%) and hexadecyl trimethyl ammonium chloride (CTAC, 98.0%) were purchased from Sinopharm Chemical Reagent Co., Ltd. The water used in all experiments was deionized. All the chemical reagents were used as received without further purification. Synthesis of Au rods High-quality Au rods encircled by {100} and {110} facets were prepared through a modified seed-mediated growth process [42] . In the preparation of seed solution, an aqueous solution of CTAB (0.2 M, 2.25 mL) was mixed with 2.25 mL of 0.5 mM HAuCl 4 , and kept stirring in a 20 mL glass vessel. Subsequently, 157.5 μL ice-cold aqueous solution of NaBH 4 (16.4 mM) was quickly added. Then the seed solution was kept vigorous stirring, resulting in the formation of a brownish yellow solution. After stirring for 1 min, it was kept at 30 °C for 30 min before further use. In a typical synthetic process of Au rods, 195 mL CTAB (0.1 M) was kept in a 250 mL conical flask under magnetic stirring at room temperature. Subsequently, 5 mL aqueous solution of HAuCl 4 (20 mM) and 5 mL aqueous solution of AgNO 3 (4 mM) were injected into the conical flask successively. Then the aqueous solutions of AA (0.1 M) were dropped into the above solution until the color of the solution turned from orange to colorless. After another 300 μL AA (0.1 M) was added, 1 mL prepared seed solution was quickly added into the flask with a pipette. After reaction for 1 h, the products were centrifuged with deionized water for three times at 11,000 rpm for 10 min. The precipitation was dispersed in deionized water and measured by inductively coupled plasma mass spectrometry (ICP-MS) for further use. Synthesis of Au rod@CuPd 2 The co-deposition of Cu and Pd atoms on Au rod was achieved via an epitaxial growth method. In a typical synthetic process for Au rod@CuPd 2 sample, 70.8 mL aqueous solution containing 0.1 M hexadecyl trimethyl ammonium chloride (CTAC) was kept in a 100 mL round-bottom flask under magnetic stirring at 50 °C, followed by the addition of a suspension containing 4 mg Au rods. Then the aqueous solutions of K 2 PdCl 4 (1 mL, 10 mM) and CuCl 2 (1 mL, 10 mM) were added into the flask. Subsequently, 2.4 mL aqueous solution of ascorbic acid (0.1 M) was added into the flask with a pipette immediately. After reaction for 1 h, the products were centrifuged with deionized water for three times at 9500 rpm for 10 min before being re-dispersed in 4 mL deionized water. Synthesis of Au rod@CuPd x - y Other Au rod@CuPd x - y samples were synthesized by following similar procedures except for the use of different amounts of K 2 PdCl 4 and CuCl 2 . The usage of K 2 PdCl 4 and CuCl 2 : (1) 1.2 mL K 2 PdCl 4 and 800 μL CuCl 2 for Au rod@CuPd 2.5 , (2) 1.4 mL K 2 PdCl 4 and 600 μL CuCl 2 for Au rod@CuPd 3.6 , (3) 1.6 mL K 2 PdCl 4 and 400 μL CuCl 2 for Au rod@CuPd 6.1 , (4) 1.8 mL K 2 PdCl 4 and 200 μL CuCl 2 for Au rod@CuPd 8.8 , (5) 1.9 mL K 2 PdCl 4 and 100 μL CuCl 2 for Au rod@CuPd 14.2 , (6) 200 μL K 2 PdCl 4 and 200 μL CuCl 2 for Au rod@CuPd 2 -0.1, (7) 500 μL K 2 PdCl 4 and 500 μL CuCl 2 for Au rod@CuPd 2 -0.2, (8) 1.5 mL K 2 PdCl 4 and 1.5 mL CuCl 2 for Au rod@CuPd 2 -0.9, and (9) 2.0 mL K 2 PdCl 4 and 2.0 mL CuCl 2 for Au rod@CuPd 2 -1.2. In situ NAP-XPS characterization In situ NAP-XPS was performed at the X-ray Photoelectron Spectroscopy and UV Photoelectron Spectroscopy Endstation (BL24A1) in the National Synchrotron Radiation Center (NSRRC). The apparatus was composed of three chambers, including a sample load-lock chamber, a preparation chamber and an analysis chamber. The analysis chamber was equipped with an SPEC Phoibos 150 energy analyzer. The catalyst was dropcast onto a clear silicon wafer, and dried at room temperature. The samples were then loaded into the load-lock chamber and delivered to preparation chamber for 10 min Ar ion sputtering treatment. High-purity CO 2 (99.9999%) was introduced into the analysis chamber with the partial pressure maintained at 0.25 mbar. Afterwards, the samples were delivered to the analysis chamber. NAP-XPS were recorded with 1170 eV photons while a Xe lamp source (PLS-SXE300D, Beijing Perfectlight) was used as a light source. The Cu 2 p , Pd 3 d and C 1 s spectra were recorded continuously for 1 h and light illumination was introduced into the analysis chamber in the middle 30 min. The incident photon energy was calibrated against Au 4 f core level measured with an Au foil mounted beside the sample. Sum frequency generation vibrational spectroscopy characterization We performed the offline SFG-VS study on Au rod@CuPd 2 with a home-built SFG-VS spectrometer. Briefly, an 1 kHz Ti:Sapphire laser amplification system (Spitfire Ace, Spectra-Physics) was employed to produce a ~80 fs pulse with the center wavelength at 800 nm and a pulse energy of 6 mJ. About 3 mJ of this output was fed into an optical parametric amplifier (TOPAS Prime, Light Conversion) to generate the femtosecond broadband infrared (IR) pulse, while another portion of the 800 nm fundamental beam (~1.2 mJ) was guided into a 4f pulse shaper to produce the narrowband upconversion pulse centered around 800 nm with a FWHM of ~7 cm −1 . The broadband IR and narrowband upconversion pulses overlapped at the sample surface both spatially and temporally with their incident angles fixed at 45° and 63° against the surface normal, respectively. The sum frequency generation signals were acquired in a reflective geometry with a high-resolution optical spectrometer (SR-500i-A, Andor Inc.) coupled with a CCD detector (Du970P-BVF, Andor Inc.). Before the SFG-VS measurements, the sample films were deposited on the flat side of a CaF 2 half cylinder support and washed with water vapor for 20 min to totally remove the hydrocarbon surfactant. The newly prepared films were transferred into CO 2 -saturated ultrapure water environment enclosed by a Teflon vessel, followed by the exposure to the broadband irradiation (Xe lamp) for 20 min. During the offline SFG-VS experiment, the averaged pulses of IR and upconversion pulses were kept at 3.0 and 9.0 μJ, respectively, for Au rod@CuPd 2 at ppp (p-SFG, p-Vis, and p-IR) and ssp (s-SFG, s-Vis, and p-IR) polarization to avoid any surface damage. All SFG signals were averaged for 600 k shots. Characterization Transmission electron microscopy (TEM) images were taken on a Hitachi Model H-7700 microscopy at an accelerating voltage of 100 kV. High-resolution transmission electron microscopy images and energy dispersive spectroscopy mapping profiles were recorded on a JEOL ARM-200F field-emission transmission electron microscope at an accelerating voltage of 200 kV. Powder XRD patterns were collected using a Japan Rigaku DMax-γA rotating anode X-ray diffractometer equipped with diffracted beam graphite monochromator (Cu Kα radiation (λ = 1.54178 Å)). The concentrations of various elements in the prepared samples were measured with a Thermo Scientific PlasmaQuad 3 inductively-coupled plasma mass spectrometry (ICP-MS) after dissolving them with a mixture of HCl and HNO 3 (3:1, volume ratio). Ultraviolet-visible (UV-Vis) extinction spectra were recorded in the spectral region of 300–1000 nm with an Agilent Technologies Cary 60 spectrometer. The samples were diluted with deionized water to the same concentration before being measured in a quartz cuvette. Photocatalytic CO 2 reduction reaction measurements The light-driven catalytic CO 2 RR was performed in a homemade quartz tube. Typically, 1 mg catalyst sample (based on inductively coupled plasma mass spectrometry, ICP-MS measurements) was dispersed in deionized water (18.25 MΩ cm) in the tube to reach a total suspension volume of 4 mL, which was then vacuumed and saturated with high-purity CO 2 (99.9999%) for three times and sealed with a glass stopper after filled with 1 atm high-purity CO 2 (99.9999%). Subsequently the suspension was vigorously stirred, and illuminated using a Xe lamp source (PLS-SXE300D, Beijing PerfectLight) at a light intensity of 400 mW cm –2 (full-spectrum light). The resultant reaction gas was then analyzed by gas chromatography (GC, 7890 A, Agilent) equipped with a flame ionization detector (FID). The control experiments in dark environment were performed under the same conditions except the exclusion of light with an aluminum foil or the exclusion of carbon dioxide with high-purity Ar (99.9999%). Photocatalytic CO 2 reduction measurements in a gas-solid biphase reactor The light-driven catalytic CO 2 RR was performed in a 10 cm diameter spherical reactor equipped with a 1 cm diameter quartz window as the light inlet. The inside of the spherical reactor was uniformly coated with foamed polytetrafluoroethylene, whose reflectance is 0.978, 0.991, 0.989 and 0.988 at 400, 600, 800 and 1000 nm, respectively. Typically, 0.5 mg catalyst sample (based on ICP-MS measurements) was dispersed evenly on a 3 cm diameter quartz wool sheet, which was then gently dried in an inert atmosphere and installed in the center of the integrating sphere reactor facing the light inlet. Subsequently, 0–0.4 mL CO 2 -saturated water was dropped on the quartz wool sheet. After the reactor was sealed with the quartz window, high-purity CO 2 (99.9999%) was introduced to purify the reactor and filled to 0–2 atm. Then a Xe lamp source (PLS-SXE300D, Beijing PerfectLight, 400 mW cm –2 , full spectrum) was employed as a light source to irradiate the catalyst from the light inlet. The resultant reaction gas was then analyzed by gas chromatography (GC, 7890 A, Agilent) equipped with a FID. The control experiments in dark environment were performed under the same conditions except the exclusion of light with an aluminum foil or the exclusion of CO 2 with high-purity Ar (99.9999%). Computational details DFT calculations with periodic boundary conditions (PBC) were carried out using the program ADF-BAND 2019. Perdew-Burke-Ernzerhof exchange-correlation functional with DFT-D3 (BJ) dispersion correction and TZP basis set incorporated with ZORA approach to include the scalar relativistic effects were employed under the spin-unrestricted scheme. A 5 × 5 slab with three atomic layers was used to mimic the Pd (100) surface with Cu doping. During the geometry optimizations, only the top layer was relaxed and the two bottom layers were frozen at the bulk positions. A 3 × 3 × 1 k -point grid was used to sample the first Brillouin zone under the two-dimensional PBC. A \(\varGamma\) -only k -mesh was adopted in the energy decomposition analysis for extended systems (pEDA) with the extension of natural orbitals for chemical valence. Since the strong interaction of photons and plasmonic metal can result in an alternating electric field, which is localized near the metal surface following the law of sines ( E = A sin t , where E , A and t represent electric field intensity, amplitude and time, respectively). In order to investigate the influence of the electric field induced by LSPR on the adsorbed molecules, the adsorption energy and bond length of these molecules were simulated under specific electric field conditions. Given the monotonicity and periodicity of the sine function, the three most representative conditions were studied. Specifically, when t = 0 or π, t = π/2 and t = 3π/2, and A = 0.04 au, the E values are 0, 0.04 and −0.04 au, respectively. Taken together, the external electric fields with the directions pointing toward/away the substrate were applied in simulations considering the field created from surface plasmon polariton.